Catch-bond behaviour facilitates membrane tubulation by non-processive myosin 1b Myosin 1b is a single-headed membrane-associated motor that binds to actin filaments with a catch-bond behaviour in response to load. In vivo , myosin 1b is required to form membrane tubules at both endosomes and the trans-Golgi network. To establish the link between these two fundamental properties, here we investigate the capacity of myosin 1b to extract membrane tubes along bundled actin filaments in a minimal reconstituted system. We show that single-headed non-processive myosin 1b can extract membrane tubes at a biologically relevant low density. In contrast to kinesins we do not observe motor accumulation at the tip, suggesting that the underlying mechanism for tube formation is different. In our theoretical model, myosin 1b catch-bond properties facilitate tube extraction under conditions of increasing membrane tension by reducing the density of myo1b required to pull tubes. Understanding the mechanisms that cells use to produce physical forces to control their own shape and the morphology of their compartments is a fundamental problem of cell biology. Because of their ability to pull on membranes and transport vesicles or organelles [1] , [2] , microtubule-associated motor proteins are key factors in membrane remodelling [3] . Indeed, in vitro , these motors can pull membrane tubular networks along microtubules from Golgi or endoplasmic reticulum membranes [4] , [5] , [6] . In addition, processive motors, that is, motors making multiple consecutive steps on their cytoskeleton substrate, such as kinesin-1, are able to cooperatively extract nanotubes along microtubules by exerting a force on the membrane to which they are bound [7] , [8] , [9] . Growing evidence indicates that actin-based motors, such as myosins 5b, 6 and 1b, are also involved in membrane tubule formation in vivo [10] , [11] , [12] , [13] . We previously reported that myosin 1b (myo1b), although non-processive, that is, it detaches from actin filament during each ATPase cycle and makes a single step only, is indispensable for the formation of post-Golgi tubular carriers from the trans-Golgi network (TGN) and modulates the membrane tube extension from sorting endosomes [12] , [13] . Similar to the other members of the myosin 1 family, myo1b is a membrane-associated single-headed motor that binds membrane via its carboxy terminal domain also named tail. This region presents a highly basic tail homology 1 (TH1) domain that targets myosins 1 to lipid membranes and a pleckstrin homology motif in the TH1 domain that targets myo1b to the membrane containing phosphatidylinositol-4,5-bisphosphate (PI(4,5)P 2 ) [14] , [15] . Myosins 1 are non-processive but some members of this family, including myo1b, have a catch-bond behaviour (a decreasing detachment rate on increasing load) [16] , [17] , [18] in contrast, for example, to kinesin-1, which has a slip-bond behaviour (an increasing detachment rate with increasing load) [19] . Despite the crucial role of myo1b in tubule formation established in vivo , the understanding of the mechanism by which a single-headed, non-processive and force-sensitive motor contributes to the tubule formation is lacking. Two fundamental questions can be raised: (i) is myo1b able and sufficient to pull membrane tubes along actin filaments? (ii) more generally, how can a non-processive motor elongates a membrane tube? Here we show using a reconstituted system that myo1b can extract tubes from giant unilamellar vesicle (GUV) containing PI(4,5)P 2 . We propose a theoretical model that emphasizes the importance of myo1b catch-bond properties for facilitation of tube extraction. Myo1b elongates tubes from GUVs We first reconstituted a minimal system composed of purified full-length recombinant myo1b, GUV containing PI(4,5)P 2 as a model membrane and actin filaments (F-actin) bundled with a uniform polarity on a glass substrate as tracks for myo1b ( Fig. 1 ). Instead of artificially binding molecular motors to GUVs via biotin–streptavidin coupling as it was previously done with kinesins or NCD, we took advantage of myo1b biologically relevant interactions with PI(4,5)P 2 lipids and bound the full-length motor with GUVs via these lipids. 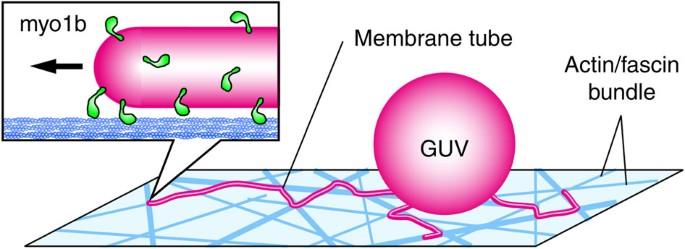Figure 1:Scheme of the reconstitutedin vitrosystem. Membrane tubes grow from a giant unilamellar vesicle (GUV) coated with myosins 1b (myo1b) sedimented on actin filaments bundled by fascin immobilized on a glass substrate. Figure 1: Scheme of the reconstituted in vitro system . Membrane tubes grow from a giant unilamellar vesicle (GUV) coated with myosins 1b (myo1b) sedimented on actin filaments bundled by fascin immobilized on a glass substrate. Full size image We produced and purified recombinant myo1b using the Flp-In system [13] that allows to obtain proteins on a large scale from mammalian cell culture (Methods). Analysis by gel electrophoresis of purified myo1b demonstrated a strong enrichment in myo1b ( Supplementary Fig. 1 ). The analysis by cryo-EM of the preparation showed isolated molecules of 27 nm length on average as previously reported for myo1b [20] ( Fig. 2a ). We also found myo1b bound to rare native vesicles present in the preparation ( Fig. 2b ), demonstrating the capacity of myo1b to bind membranes in vivo . Moreover, the motor property of recombinant myo1b was preserved after purification and fluorescent labelling, as judged by F-actin gliding motility assays. Fluorescent myo1b was able to move fluorescent F-actin at room temperature (RT) and in the presence of 2 mM ATP with an average velocity of 56.0±4.3 nm s −1 ( Supplementary Fig. 2 ), in the same range as those previously reported for myo1b [21] . We next investigated the ability of myo1b to bind small liposomes in a fluid phase, generated from a lipid film composed of egg yolk L -α-phosphatidylcholine (egg PC), cholesterol and in the presence or the absence of PI(4,5)P 2 . Analysis by cryo-EM revealed that myo1b bound to the liposomes containing PI(4,5)P 2 ( Fig. 2c and Supplementary Fig. 3A versus B ). Although myo1b molecules were densely distributed, forming a brush-like structure, no clustering of the motors was observed at the surface of the liposomes ( Fig. 2c ; Supplementary Fig. 3B and C ). Overall, these data showed that purified myo1b was functional and able to interact with the PI(4,5)P 2 -containing membrane. 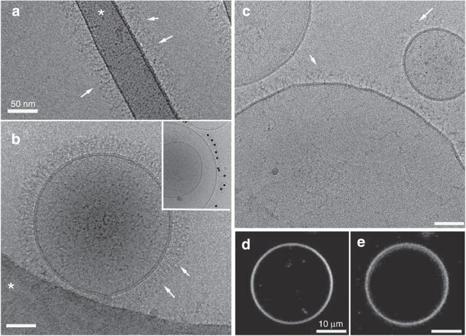Figure 2: Purified myo1b binds small and giant liposomes. (a) Cryo-EM image of myo1b (white arrows pointing to the head groups). The dark network is the carbon of the holey EM grid. (b) Cryo-EM image of one of the rare native vesicles copurified with myo1b. Myosin heads point 27 nm outwards the lipid bilayer. (Inset) Immunolabelling of myo1b bound to native vesicles. (c) Cryo-EM image of myo1b bound on a small synthetic liposome made of egg PC/cholesterol/PI(4,5)P2incubated with purified recombinant myo1b. Despite the high protein density, no myosin cluster is observed. (d,e) Confocal microscopy image of myo1b bound to a PI(4,5)P2-containing GUV. Labelling corresponds to (d) 0.3% Texas Red DHPE (mol/mol) and (e) Alexa Fluor 488 conjugated myo1b. Scale bars, (a–c) 50 nm, (d,e) 10 μm. White arrows: equatorially bound myosins. White star: carbon network of the holey grids. Figure 2: Purified myo1b binds small and giant liposomes. ( a ) Cryo-EM image of myo1b (white arrows pointing to the head groups). The dark network is the carbon of the holey EM grid. ( b ) Cryo-EM image of one of the rare native vesicles copurified with myo1b. Myosin heads point 27 nm outwards the lipid bilayer. (Inset) Immunolabelling of myo1b bound to native vesicles. ( c ) Cryo-EM image of myo1b bound on a small synthetic liposome made of egg PC/cholesterol/PI(4,5)P 2 incubated with purified recombinant myo1b. Despite the high protein density, no myosin cluster is observed. ( d , e ) Confocal microscopy image of myo1b bound to a PI(4,5)P 2 -containing GUV. Labelling corresponds to ( d ) 0.3% Texas Red DHPE (mol/mol) and ( e ) Alexa Fluor 488 conjugated myo1b. Scale bars, ( a – c ) 50 nm, ( d , e ) 10 μm. White arrows: equatorially bound myosins. White star: carbon network of the holey grids. Full size image We next analysed the formation of tubes on GUVs by optical microscopy. Two hundred nanomolars of myo1b was then incubated with GUVs, generated by electroformation from lipid films with the same composition as that of the small liposomes, supplemented with 0.3% Texas Red 1,2-dihexadecanoyl-sn-glycero-3-phosphoethanolamine (Texas Red DHPE) (mol/mol). In all, 10–20% of the GUVs showed a homogeneous fluorescence that does not result from the interaction of free fluorescent dye with the membrane ( Supplementary Fig. 4 ) but was due to myo1b binding ( Fig. 2d,e ). Furthermore, no binding was found in the absence of PI(4,5)P 2 ( Supplementary Figs 3A and 5 ). We prepared F-actin bundled with fascin, leading to polar bundles. After sedimentation of GUVs covered with myo1b on F-actin bundles randomly fixed on a poly- L -lysine-coated glass slide, we monitored tube extension at the bottom of the GUVs in contact with the actin bundles using confocal microscopy. We observed membrane tube growth along F-actin bundles in the presence of ATP ( Fig. 3a and Supplementary Movie 1 ). Myo1b, membrane and F-actin were co-localized as shown by fluorescence microscopy ( Fig. 3b ). Tubes do not grow by passive spreading of the membrane decorated with myo1b on F-actin since replacement of 2 mM ATP by 2 mM ADP inhibited extraction ( Supplementary Fig. 6 ). Myo1b ATPase activity and its catch-bond property are regulated by calcium concentration, as calcium releases calmodulin—a regulatory myosin light chain—from myo1b [21] , [22] . In agreement with these reports, we observed that complementing our assay with 0.5 mM calcium (in the absence of EGTA) totally inhibited tube extraction ( Fig. 4a ). Furthermore, addition of 2 mM calcium (in the presence of 1 mM EGTA) during tube extension induced fast retraction ( Fig. 4b ). The effect was not due to an osmotic shock. The osmolarity of the calcium solution was carefully adjusted to the same value as the assay buffer. Moreover, the distribution of fluorescent myo1b remained homogeneous on calcium addition ( Supplementary Fig. 7 ), although calcium is known to cluster PI(4,5)P 2 in certain conditions [23] , [24] . This demonstrates that active myo1b are responsible for tube growth. 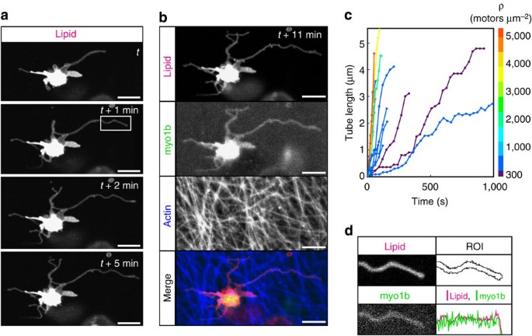Figure 3:Myo1b pulls membrane tubes from a PI(4,5)P2-containing GUV along F-actin bundles. (a) Growth of membrane tubes between a reference time t (top) and t+5 min (bottom) followed with confocal microscopy. Confocal sections at the bottom of the GUV where the GUV is in contact with the substrate covered with actin bundles are shown. Zoom of the box is shown ind. (b) Images of the same tube at t+11 min showing the distribution of lipid (magenta), myo1b (green) and actin (blue) (c) Growth kinetics of membrane tubes as a function of myo1b total density (actin bundle-bound and - unbound motors). Motor density is represented according to the colour scale represented on the right. Data at low density are binned over three points. (d) Zoom of the tip of the tube (box ina) showing confocal fluorescence microscopy images (left) and intensity profiles (bottom right) of lipid membrane and myo1b. Scale bars, 5 μm. Figure 3: Myo1b pulls membrane tubes from a PI(4,5)P 2 -containing GUV along F-actin bundles. ( a ) Growth of membrane tubes between a reference time t (top) and t+5 min (bottom) followed with confocal microscopy. Confocal sections at the bottom of the GUV where the GUV is in contact with the substrate covered with actin bundles are shown. Zoom of the box is shown in d . ( b ) Images of the same tube at t+11 min showing the distribution of lipid (magenta), myo1b (green) and actin (blue) ( c ) Growth kinetics of membrane tubes as a function of myo1b total density (actin bundle-bound and - unbound motors). Motor density is represented according to the colour scale represented on the right. Data at low density are binned over three points. ( d ) Zoom of the tip of the tube (box in a ) showing confocal fluorescence microscopy images (left) and intensity profiles (bottom right) of lipid membrane and myo1b. Scale bars, 5 μm. 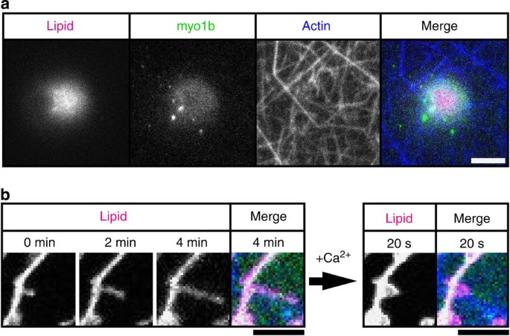Figure 4: Calcium strongly affects tube growth. (a) Calcium prevents myo1b from extracting tubes: confocal microscopy images of lipid (magenta), myo1b (green) and actin (blue) at the bottom of a GUV in the presence of 0.5 mM calcium. No tube extraction was observed. (b) Addition of calcium induces retraction from a growing tube: confocal microscopy images of lipid (magenta), myo1b (green) and actin (blue) during tube growth (left) and 20 s after the addition of 2 mM calcium (right). Note that tube retraction is much faster than tube extension. Scale bar, 5 μm. Full size image Figure 4: Calcium strongly affects tube growth. ( a ) Calcium prevents myo1b from extracting tubes: confocal microscopy images of lipid (magenta), myo1b (green) and actin (blue) at the bottom of a GUV in the presence of 0.5 mM calcium. No tube extraction was observed. ( b ) Addition of calcium induces retraction from a growing tube: confocal microscopy images of lipid (magenta), myo1b (green) and actin (blue) during tube growth (left) and 20 s after the addition of 2 mM calcium (right). Note that tube retraction is much faster than tube extension. Scale bar, 5 μm. Full size image Tube elongation velocity and myo1b density along the tubes were determined using time-lapse confocal microscopy (Methods). Myo1b density on the membrane has been measured from fluorescence analysis on the tubes (Methods). Remarkably, although myo1b is non-processive, directional tube growth was observed with myo1b densities of the same order of magnitude as the threshold density for processive (kinesin-1) or non-processive (NCD) kinesins (as low as 300 motors μm −2 ) [9] , [25] , [26] . Myo1b-associated tubes grew regularly with an average velocity ranging from 5 to 100 nm s −1 (typical elongation plots are shown in Fig. 3c ) with myo1b density ranging from 300 motors μm −2 to 5,200 motors μm −2 (see below and Supplementary Movies 1–3 ). Furthermore, Myo1b did not accumulate at the tube tip ( Fig. 3d ) in contrast to kinesins pulling tubes [9] , [25] . Finally, in contrast with NCD [25] , we never observed bidirectional growth of the tubes. This suggests different underlying mechanisms of tube formation for single-headed non-processive myosins and processive or non-processive kinesins, and thus requires the development of a new theoretical model to understand this process. Myo1b catch-bond behaviour facilitates tubule elongation Our theoretical model makes the following hypotheses (see Fig. 5a for a sketch): (i) myo1b remains attached to the membrane due to its high affinity K d =6 nM (ref. 15 ); its detachment rate is insensitive to load in the range of forces investigated and thus neglected; myo1b diffuses along the tube surface and binds transiently to F-actin during the ATPase cycle. Thus, binding/unbinding refers only to myo1b and F-actin, but not to myo1b and membrane. (ii) As the membrane is fluid, myo1b exerts a force only at the tube tip [9] . (iii) Being non-processive, myo1b performs only one step after binding to F-actin; membrane tube extension requires, therefore, the binding of another motor ahead of the leading motor; yet myo1b being a catch-bond motor, its binding time increases with increasing load. Thus, tube dynamics results from binding and unbinding kinetics of the tip motor. The growth is facilitated by an increase in myo1b density and by applying a load on the myo1b. The unbinding rate of the catch-bond myo1b from actin filaments ω off decreases exponentially with load f ω off ( f )=1.6exp(− f . d det / k B T )+0.02 s −1 with, k B T / d det =0.3 pN [17] (Fig. 5a ) (see details on the microscopic model for myo1b ATPase cycle in Supplementary Note ). In the following, we use ω off as ω off (0). We call n f the number of filaments in the actin bundle accessible to the myo1b motors, which corresponds to a fraction of the total number. Motor binding on F-actin is possible if one of the n f filaments of the actin bundle is not already occupied. We write the binding rate as where d ≈5 nm is the motor step, R 0 is the membrane tube radius and ρ b the surface density of bound motors. We suppose here that the binding rate of an isolated motor on a single filament ω on ( Fig. 5a ) is independent of applied load f . The unbound motors of surface density ρ u diffuse along the tube with a diffusion constant D ( Fig. 5a ), whereas the bound motors of density ρ b perform their powerstroke before unbinding. 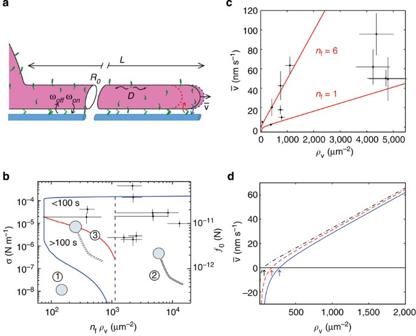Figure 5:Theoretical modelling and comparison with experimental data. (a) Sketch of the model withDthe diffusion coefficient of the motors (green) on the membrane (magenta),the tube growth velocity,ωon/ωoffthe binding/unbinding rates of motors on the actin bundle andR0the tube radius. The motors bound at the tip support the load on the tube. The tube lengthLincreases by one step (blue dashed line) if a motor binds (blue arrow) further on the actin bundle (blue). If the last motor bound at the tip unbinds (red arrow), the tube retracts until it reaches a bound motor (red dashed line). (b) Phase diagram of tube extraction as a function of membrane tensionσ(or equivalently the plateau forcef0, asσ=1/2κ(f0/2π)2) and the motor density on the vesicleρvrescaled with the number of F-actin in the bundlesnf(seeSupplementary Note) (n=11). In the region 1, no tube is pulled (circle). In 2, tubes are systematically extracted (circle+tube). In 3, tubes are extracted stochastically. 3 is subdivided in two parts, corresponding to extraction time larger or lower than 100 s. Experimentally observed tubes (black crosses) are in 2 or in the ‘fast’ region 3. (c) Growth velocityversusρv(deduced fromSupplementary equation (4))from experiments (n=12). Error bars representSD× 0.67, corresponding to 50% confidence interval (see Supplementary for details on error bars). The experimental points are bound by the theoretical curves (equation (2)) (red) with the catch-bond activated,ρv=ρuandnf=1 and 6. (d) Theoretical variation ofversusρv(Eq. (2)) for three different forcesf=0 (blue), 0.3 (red) and 1 pN (black), andnf=4. The arrows correspond to the respective motor density thresholds. The kinetic equations for a tube advancing at velocity are: Figure 5: Theoretical modelling and comparison with experimental data . ( a ) Sketch of the model with D the diffusion coefficient of the motors (green) on the membrane (magenta), the tube growth velocity, ω on / ω off the binding/unbinding rates of motors on the actin bundle and R 0 the tube radius. The motors bound at the tip support the load on the tube. The tube length L increases by one step (blue dashed line) if a motor binds (blue arrow) further on the actin bundle (blue). If the last motor bound at the tip unbinds (red arrow), the tube retracts until it reaches a bound motor (red dashed line). ( b ) Phase diagram of tube extraction as a function of membrane tension σ (or equivalently the plateau force f 0 , as σ =1/2κ( f 0 /2π) 2 ) and the motor density on the vesicle ρ v rescaled with the number of F-actin in the bundles n f (see Supplementary Note ) ( n =11). In the region 1, no tube is pulled (circle). In 2, tubes are systematically extracted (circle+tube). In 3, tubes are extracted stochastically. 3 is subdivided in two parts, corresponding to extraction time larger or lower than 100 s. Experimentally observed tubes (black crosses) are in 2 or in the ‘fast’ region 3. ( c ) Growth velocity versus ρ v (deduced from Supplementary equation (4)) from experiments ( n =12). Error bars represent SD × 0.67, corresponding to 50% confidence interval (see Supplementary for details on error bars). The experimental points are bound by the theoretical curves (equation (2)) (red) with the catch-bond activated, ρ v = ρ u and n f =1 and 6. ( d ) Theoretical variation of versus ρ v (Eq. (2)) for three different forces f =0 (blue), 0.3 (red) and 1 pN (black), and n f =4. The arrows correspond to the respective motor density thresholds . Full size image In our experiments, we only measure the total density ρ = ρ b + ρ u . Our model predicts that ρ is constant if (with r = ρ b/ ρ ) and t* larger than 10 3 s in our experimental conditions ( Supplementary Note ). Therefore, the surface density on the vesicle ρ v is equal to the density along the tube, ρ v = ρ u ( Supplementary Note ). Moreover, in agreement with our observations no extended motor accumulation at the tip as observed for tubes pulled by kinesins is expected. In the Supplementary Note , we model the elongation of the tube as a Markov process with advancing and receding steps. The elongation velocity reads: where P (1) is the probability to find a single motor at the tip. The first term is the advancing velocity due to the binding of new motors elongating the tube by d , whereas the second term is the retraction velocity due to the unbinding of the first motor ( Supplementary Note ). The retraction step is d /1− q where because the tube retracts until another bound motor sustains the force. The elongation velocity decreases with decreasing motor concentration and vanishes at . Because of the catch-bond effect, the critical density decreases with the membrane force, by a factor 10 for a few pN force. We next determined the conditions for tube extraction that we summarized in the phase diagram of Fig. 5b . The force required to pull a tube from a vesicle increases linearly with the amplitude of the vesicle deformation and reaches a plateau when the tube is formed [27] . The plateau force f 0 and the radius R 0 depend on the membrane bending modulus κ and the vesicle tension σ , f 0 =2π(2 σκ ) 1/2 and R 0 =( κ /(2 σ )) 1/2 (ref. 27 ). If the motor density on the vesicle is larger than the critical density at vanishing force , myo1b systematically extracts a tube ( Fig. 5b , region 2). If the motor concentration is such that , tubes do not have a positive velocity at vanishing force. Thus, no tube extraction occurs until fluctuations of motors binding to F-actin produce a membrane deformation sufficient to initiate tube elongation. By analogy with a particle in a metastable energy well, we describe this region of the phase diagram as stochastic extraction ( Fig. 5b , region 3). In this regime, we calculated the average time for tube extraction as a first passage problem ( Supplementary Note ). Finally, if , no tube is extracted ( Fig. 5b , region 1). In region 3 characteristic of catch-bond, we distinguish two subregions depending on whether the average extraction time is larger or smaller than the experimental time 100 s (region 3, Fig. 5b ). We consider that the probability of extraction vanishes if the extraction time is larger than 100 s. The experimental conditions under which tubes are extracted are well supported by the calculated phase diagram ( Fig. 5b ). As demonstrated in ref. 27 , the force to pull a tube can be calculated from the membrane bending rigidity and tube radius, regardless of the vesicle morphology, as the theory was developed for a patch of membrane. Consequently, both the plateau force and the membrane tension for each tube were calculated from and where the radius R 0 was deduced from fluorescence analysis (Methods) and κ from independent measurements κ=31.7±3.0 k B T =127±12 pN nm (Methods and Supplementary Fig. 8 ). As the unbinding rate is expected to increase when exceeding a force f m (ref. 28 ), in agreement with experiments, we set f m =35 pN. No tube can be extracted under these conditions ( Fig. 5b , region 1). All vesicles generating tubes in our experiments correspond to region 2 of spontaneous tube growth of the phase diagram or to subregion 3 (average extraction time smaller than 100 s). In region 2, several tubes can be extracted from the same GUV, whereas in region 3 only one tube is extracted ( Fig. 5b and Supplementary Movie 2 ). We then compared theory and experimental data for the growth velocity as a function of the motor density on the vesicle ρ v . Experimentally, we can measure the protein density on the tube ρ and the tube radius R 0 ; the density ρ v is calculated by solving Supplementary equation (4) (see Supplementary Note ). As predicted by using equation (2), the experimental mean velocity increases with density ( Fig. 5c ) and even exceeds the velocity of a free F-actin gliding on myo1b (See Supplementary Note for more details). The number of actin filaments in the bundles involved in tube growth cannot be directly measured. With ω on =1.5 × 10 −3 μm 2 s −1 , we found that n f ranges between 1 and 6 in our samples ( Fig. 5c ), a narrow range in agreement with ref. 29 , which is consistent with our assumption that ω on is independent of applied force. The binding rate for a membrane saturated with motors is on the order of a few s −1 , in agreement with the phosphate release rate measured in ref. 17 . We plotted the theoretical variation of the tube velocity versus ρ v to evaluate the effect of catch-bond on the critical density . On the basis of our experiments, we used the median value n f =4 for this plot ( Fig. 5d ). Because of the catch-bond effect, decreases from 280 to 22 μm −2 ; for f >3pN, the velocity becomes independent of force. According to this plot, the minimum density of catch-bond motor per accessible filament to form tubes corresponds to about 10 myo1b bound to 100 nm radius endosomes. This quantity is in the same range as the number of proteins that have been measured at the surface of a synaptic vesicle [30] . In conclusion, our theoretical model accounts for our experimental data and highlights the importance of myo1b catch-bond property for its in vivo function. Our results demonstrate for the first time that a myosin-1 has the capacity to tubulate membrane along F-actin bundles at physiological density due to its catch-bond behaviour. Membrane-pulling processes rely on the specific mechanical properties of the motors. For processive kinesins, less than 10 motors at the tip are involved in tube pulling against forces up to 30 pN [31] , and growth occurs at low motor density on the membrane. In contrast, membrane tubulation by the non-processive kinesin NCD requires a high density of motors to pull tubes against the same range of forces [9] , [25] , [26] , whereas myo1b pulls at low motor density (see phase diagram, Fig. 5b ). In addition, NCD motors exhibit periods of backward motion while tubes pulled by myo1b advance at constant velocity always in the same direction. Our theoretical model predicts that these differences are due to myo1b catch-bond properties. According to this model, the formation of stochastic clusters on the tube and at its tip is not required for myo1b unlike for NCD [25] , [26] , and the number of myosins at the tip should be small (less than 10). A possible future challenge will be to investigate whether other classes of motor with different mechanical properties can pull membrane tubes. KIF1A is an interesting candidate [32] : it is very inefficient as a single molecule but can overcome much higher force than conventional kinesin when self-organized in clusters, and thus being well-adjusted to pulling membrane tubes against high load [33] . Our observations indicate that bundling of F-actin facilitates tube pulling by myo1b, by decreasing the threshold density of motors on the membrane. This raises the question regarding the organization of the F-actin network (branched or bundled) available in the TGN region in vivo. A population of short and branched F-actin, revealed by a tropomyosin isoform, was observed close to Golgi membranes by electron microscopy [34] ; moreover, Arp2/3-dependent F-actin structures are associated with the base of membrane tubules that exit from the TGN [13] . Nevertheless, the formin mDia1, which stimulates actin nucleation and actin bundle elongation, participates also in the formation of carrier vesicles in this region [35] . Both actin organizations being present at the TGN, the next question will be therefore to identify the organization used by myo1b in this region. In cells, both microtubule-associated motors and myosins are involved in membrane tubule formation and elongation from the trans-Golgi network [4] , [5] , [6] , [13] . We propose that myo1b acts prior to microtubule-associated motors in the formation of tubular-carrier precursors. Myo1b and F-actin being closely associated to the membrane compartment may first pull small tubes that will then reach microtubules and allow kinesins to relay myosins for tubule elongation. Myosins and F-actin would thus bridge the gap between cell membranes and microtubules. Reagents Alexa Fluor 488 5-SDP ester, Alexa Fluor 594 phalloidin, Texas Red 1,2-dihexadecanoyl-sn-glycero-3-phosphoethanolamine (Texas Red DHPE), Alexa Fluor 647 conjugated actin from rabbit muscle, non-labelled phalloidin and streptavidin-coated bead were purchased from Life Technologies. LabSafe GEL Blue was from G-Biosciences. Non-labelled actin from rabbit skeletal muscle was purchased from Cytoskeleton. L -α-phosphatidylcholine from the chicken egg (egg PC), L -α-phosphatidylinositol-4,5-bisphosphate (PI(4,5)P 2 ) from the porcine brain, cholesterol and 1,2-distearoyl-sn-glycero-3-phosphoethanolamine- N -[biotinyl(polyethylene glycol)-2000] (DSPE-PEG-biotin) were purchased from Avanti Polar Lipids. Sigillum wax was from Vitrex Medical A/S. B-PER reagent was from Pierce Chemical. Glutathione Sepharose beads, thrombin, and Superdex 200 13/300GL column were purchased from GE Healthcare. Protein A gold was kindly provided by Dr Graça Raposo (Institut Curie, UMR 144). A myo1b plasmid and an anti-myo1b antibody were prepared as described in ref. 13 . Other chemicals were purchased from Sigma Aldrich. Myo1b purification and fluorescent labelling Myo1b was purified from HEK293-Flp-In cells expressing FLAG-myo1b according to ref. 13 . More precisely, HEK293-Flp-In cells expressing FLAG-myo1b were cultured in Dulbecco’s modified Eagle medium supplemented with 10% fetal bovine serum and 0.18 mg ml −1 hygromycine in a spinner flask at 37 °C under 5% CO 2 , and collected by centrifugation (1,000 g , 10 min, 4 °C) to obtain a 4–5 g of cell pellet. The pellet was lysed in 15 ml of buffer A (30 mM HEPES at pH 7.5, 150 mM KCl, 4 mM MgCl 2 , 1 mM EGTA, 4 mM ATP, 1 mM dithiothreitol (DTT), 0.1% protease inhibitor cocktail (PIC), 1% Triton X-100) for 30 min at 4 °C and centrifuged at 3,400 g for 10 min at 4 °C. The collected supernatant was then ultracentrifuged (250,000 g , 60 min, 4 °C). The solution between pellet and floating lipid layer was carefully harvested and incubated with 150 μl of anti-FLAG beads for 2 h at 4 °C. The beads were collected by centrifugation (1,000 g , 5 min, 4 °C), washed three times with buffer A and washed once with buffer B (buffer A without Triton X-100 supplemented with 0.1% methylcellulose). FLAG-myo1b was then eluted from the beads by incubating with 0.24 mg ml −1 of 3X FLAG peptide in 300 μl buffer B for 3 h at 4 °C. After removal of the beads by centrifugation (1,000 g , 3 min, 4 °C), the protein solution was dialysed against buffer C (buffer B with 1 mM ATP) overnight at 4 °C to remove the 3 × FLAG peptide. For the in vitro tube extraction experiments, myo1b was fluorescently labelled using Alexa Fluor 488 5-SDP ester. Two microlitres of 10 mM Alexa Fluor 488 5-SDP ester in dimethyl sulphoxide was added to the protein solution after the dialysis and incubated for 8 h at 4 °C, then the solution was dialysed against buffer C overnight at 4 °C to remove free fluorescent probe. After snap freezing, the protein solution was kept at −80 °C and used during 1–2 months. The motor activity of purified and fluorescently labelled myo1b was confirmed by using F-actin gliding assay, which gave an average velocity of 56.0±4.3 nm s −1 ( Supplementary Fig. 2 ). GUV and small liposome preparation GUVs were grown from lipid films composed of 52% L -α-phosphatidylcholine from the chicken egg (Egg PC), 28% cholesterol, 20% L -α-phosphatidylinositol-4,5-bisphosphate (PI(4,5)P 2 ) and 0.3% Texas Red 1,2-dihexadecanoyl-sn-glycero-3-phosphoethanolamine (Texas Red DHPE) (mol/mol) by using the electroformation technique on ITO slides in 256 mOsm sucrose solution. With this method, we cannot predict the amount of PI(4,5)P 2 eventually incorporated into the GUVs [24] . To ensure to work at saturation of the charged density, we worked with more than 8% (mol/mol) PI(4,5)P 2 in our lipid film [24] . We obtained the largest number of GUVs binding myo1b with GUVs made from lipid films containing 20% PI(4,5)P 2 (mol/mol). The obtained GUV solution was diluted 10-fold with buffer D (30 mM HEPES at pH 7.5, 100 mM KCl, 2 mM MgCl 2 , 1 mM EGTA, 1 mM DTT, 2 mM ATP and 0.1 mg ml −1 β-casein) supplemented with glucose to adjust the osmolarity to 258 mOsm. Using optical tweezers, the bending rigidity of the GUV membrane with this composition was measured to be 31.7±3.0 k B T ( Supplementary Note and Supplementary Fig. 8 ). Small liposomes of the same composition as GUVs except Texas Red DHPE were prepared at 1 mg ml −1 lipid concentration by first drying a lipid film formed from a lipid solution and by vortexing buffer D without β-casein for 5 min in a glass vial. Small liposomes were used immediately after preparation. Cryo-electron microscopy observation Purified myo1b bound to small liposomes and purified myo1b fraction were analysed by cryo-EM. Binding of myo1b to small liposomes was achieved by incubating 200 μg ml −1 of purified myo1b with small liposomes at 0.5 mg ml −1 lipid concentration for 15 min at 4 °C before flash-freezing. A glow-discharged Quantifoil R1.2/1.3 copper grid (Quantifoil) was loaded with 5 μl of sample solution that was subsequently blotted and vitrified in liquid ethane by plunge freezing. Images were recorded under low-dose conditions with a FEI CM120 operating at 120 kV with a SSD GATAN 1k × 1k camera (Gatan Inc.) at a magnification of 35,000 resulting in 4.96 Å per pixel. The intended underfocus was set to −1.5 to −2 μm. For immunogold labelling, myo1b solution containing rare native vesicles was diluted down to 40 μg ml −1 with 30 mM HEPES at pH 7.5, 100 mM KCl and 2 mM MgCl 2 , and incubated with 1% bovine serum albumin (BSA) and anti-FLAG antibody at 20-fold dilution for 1 h at RT. Next, Protein A gold was added at 20-fold dilution. After 30 min incubation, sample was flash-frozen for cryo-EM observation. In vitro tube extraction experiments Human GST-fascin was expressed in E. coli [36] . After lysis of bacteria in phosphate buffer containing B-PER reagent GST-fascin was isolated using Glutathione Sepharose beads. Fascin was collected from the beads using 80 units of thrombin and further purified over the Superdex 200 13/300GL column. Two micromolars of Alexa Fluor 647 actin and 1.5 μM fascin were incubated in buffer E (10 mM imidazole-HCl at pH 7.5, 100 mM KCl, 1 mM MgCl 2 , 1 mM EGTA, 2 mM ATP) for 2 h at RT to form fluorescent actin/fascin bundles. Phalloidin in methanol was added at the final concentration of 24 μM and incubated for 1 h at RT to stabilize the bundles. Fluorescently labelled myo1b at 200 nM in buffer D, corresponding to 258 mOsm, and GUV solution were mixed and incubated for 30 min at 4 °C. An observation chamber was built by placing a 5-mm-thick polydimethylsiloxane block with a 6 mm diameter hole on a poly- L -lysine-coated glass slide. Forty-three microlitres of fluorescent actin/fascin bundle solution was introduced in the chamber and incubated for 10 min at RT. After removal of the bundle solution, the chamber was incubated with 100 μl of buffer D supplemented with 0.4 mg ml −1 β-casein for 5 min at RT to passivate the surface. The chamber was rinsed twice with 100 μl of buffer D. Finally, the mixture of GUV and myo1b was added to the chamber and observed at RT. Fluorescent myo1b, GUV and actin/fascin bundle were visualized through a × 63 oil immersion objective with a confocal microscope (LSM 510 Meta, Carl Zeiss). Note that quantitative parameters can be deduced from only a few % of the GUVs for the following reasons. (1) In all, 10–20% of GUVs are covered with myo1b, probably due to heterogeneity in PI(4,5)P 2 distribution. (2) In this fraction, we observe tubes arising from 10% of myo1b-covered GUVs only. (3) Only tubes that we observe growing are analysed, to be sure that they were pulled by myo1b and not due to other factors (flow in the chamber for instance). Myo1b density on tubes and tube diameter measurements The myo1b density on a membrane tube ρ and the tube diameter d tube were estimated from the fluorescence signal of the confocal microscopy images. The fluorescence intensities of myo1b ( I myo1b ) and lipid ( I lipid ) on a tube were measured after background signal subtraction. The number of myo1b molecules ( n myo1b ) corresponding to I myo1b was estimated as follows. The concentration of original myo1b solution was determined by using a BCA assay. Dilutions of the original solution were prepared at eight different concentrations ( C myo1b ). Samples containing solutions of myo1b at these dilutions were scanned by confocal microscopy at a fixed scan volume V =(scan area) × (scan depth) at three different horizontal positions and at the same height in the chamber. Parameters of the confocal microscope were set to be the same as the tube pulling experiments. The average of the fluorescence intensities of each dilution, I myo1b , was plotted versus the number of myo1b molecules, n myo1b , contained in the volume ( n myo1b = C myo1b × N A × V where N A is Avogadro constant). From the plot, we calibrate the number of myo1b from the fluorescence intensity n myo1b =α × I myo1b and measured the α constant. We then calculated n myo1b on a tube from I myo1b in the tube region. Next, the correlation between I lipid and the membrane surface area ( S lipid ) was calculated as follows. Twenty GUVs were scanned by confocal microscopy in the same conditions as the tube pulling experiments, providing circular cross-sectional images of GUVs. Each S lipid was calculated from the contour length of the GUV image multiplied by the scan depth. The β constant was deduced from the average of 20 GUVs according to S lipid = β × I lipid . The myo1b density on the tube was then derived from I myo1b and I lipid in the tube region using . The tube diameter was derived for a tube of length l as . Note that all tube diameters used when measuring motor density were smaller than the scan depth, which was typically 0.8 μm. Sequential images of fluorescent lipids were taken every 10 or 30 s during the extraction for monitoring the dynamics; the last lipid image, together with myo1b and actin fluorescence, was used for the quantitative measurements. We checked whether the bleaching of fluorescent lipids was negligible in tubes during the recording growth time. Three representative bleaching curves obtained from tube regions in different GUVs are shown in Supplementary Fig. 9 . We excluded the effect of bleaching of the lipid fluorescence since the bleaching is not significant. Membrane bending rigidity measurement A GUV with the same composition as that used in the rest of the experiments, supplemented with 0.1% (mol/mol) DSPE-PEG-biotin was partially aspirated in a micropipette. A membrane tube was extracted from the opposite side of the GUV by using a streptavidin-coated bead trapped by optical tweezers [37] . The force exerted by the bead on the membrane is given by , where κ is the membrane bending rigidity and σ is the membrane tension [27] . Thus, knowing f and σ , one can deduce κ . σ was set through the micropipette aspiration pressure ΔP , that is, the hydrostatic pressure difference between the experimental chamber and inside of the micropipette [38] . Application of Laplace law gives , where R p and R v are the pipette and GUV radius, respectively. σ was increased stepwise, and, for each step, f was calculated from the average bead displacement x − x 0 from its equilibrium position x 0 in the optical trap using the linear relationship f = k ( x − x 0 ), where k is the trap stiffness. The bead position was measured by video tracking, and k was determined by using the viscous drag method [39] . A linear fit of the data then allowed us to determine the bending rigidity κ of the GUV membrane. Supplementary Fig. 8 shows a representative data set during such a measurement. We obtained the value κ =31.7±3.0 k B T ( n =9). The error corresponds to s.d. How to cite this article: Yamada, A. et al. Catch-bond behaviour facilitates membrane tubulation by non-processive myosin 1b. Nat. Commun. 5:3624 doi: 10.1038/ncomms4624 (2014).